All-silicon spherical-Mie-resonator photodiode with spectral response in the infrared region Silicon is the material of choice for visible light photodetection and solar cell fabrication. However, due to the intrinsic band gap properties of silicon, most infrared photons are energetically useless. Here, we show the first example of a photodiode developed on a micrometre scale sphere made of polycrystalline silicon whose photocurrent shows the Mie modes of a classical spherical resonator. The long dwell time of resonating photons enhances the photocurrent response, extending it into the infrared region well beyond the absorption edge of bulk silicon. It opens the door for developing solar cells and photodetectors that may harvest infrared light more efficiently than silicon photovoltaic devices that are so far developed. Single-junction photovoltaic devices suffer from intrinsic obstacles limiting their efficiency to a top value dictated by the well-known Shockley–Queisser (SQ) limit [1] . The most fundamental limitation is given by the energy band gap of the semiconductor, which determines the minimum energy of photons that can be converted into electron–hole pairs. The development of photodiode devices on micro and nanophotonic structures has opened new possibilities over the standard technology. The impinging light is strongly confined inside those photonic structures enhancing the photocarrier generation, as it has been observed in nanowire resonators [2] , [3] and in the electrooptical response of the optical cavities [4] , [5] , [6] . Simultaneously, photoexcited carriers are generated close to the collecting electrodes, boosting the power generation in photovoltaic cells [7] , [8] , [9] , [10] , [11] . Furthermore, thanks to an increased absorption near the band gap edge, some recent works report on efficiency values beyond the SQ limit [10] , [11] . However, due to the intrinsic bulk properties of silicon, a large percentage of infrared sunlight, with energy value below the fundamental absorption edge of silicon, is still useless. To tackle this obstacle, new resonant photodiode devices must be explored. One possibility concerns developing photodiodes on high-quality-factor ( Q ) silicon resonators. Infrared photons confined in high- Q resonant devices stay in the cavity for very long times, thus increasing their probability to be absorbed. It may result in a photocurrent response enhancement even at photon energy values below the absorption edge of silicon where the absorption coefficient is extremely low. In particular, spherical semiconductor microcavities can be a good platform for processing such resonant photodiodes. Very recently, several groups have developed silicon colloids [12] , [13] that, owing to their perfect spherical topology, sustain well-defined high- Q Mie resonances allowing the development of optical microcavities [12] , and metamaterials [14] . The fabrication of rectifying junctions on such silicon micro and nanocavities would open new possibilities over those so far developed on nanowire-like devices. First, the spherical topology would allow an omnidirectional light harvesting [15] . Second, in addition to an enhanced photocurrent response above and near the band gap edge, as reported for nanowire devices [7] , [8] , [9] , [10] , [11] , the strong confinement effect appearing in high- Q optical resonances would allow IR light dwelling for a time long enough to be absorbed even beyond the absorption edge of silicon. For instance, the light trapped in a Mie mode with Q ~6 × 10 3 , for a typical wavelength of 1,100 nm, would stay in the microcavity for 3,5 × 10 −12 s, the time needed to travel a distance of 300 μm in bulk silicon (equivalent to the thickness of a standard silicon solar cell). Third, the development of electronic devices on spherical shaped particles, together with the implementation of the self-assembling methods, like those reported by Whitesides, to build up three-dimensional [16] (3D) electrically connected [17] networks, may open new avenues for cost-effective large-area processing of complex electronic architectures such as regular size photodiode systems. Very recently, p – n junction devices showing a rectifying behaviour were developed on nanometre size silicon bi-spheres [18] . In this paper, we report on the development of a photodiode in a micrometre scale polysilicon sphere. The distinctive points of our work are the following: First, the impinging light couples to the resonant modes of the microcavity, resulting in a unique photocurrent response, mimicking the Mie modes of an optical resonator. Second, both the residual absorption tail of polysilicon and the high- Q values of the microcavity resonating modes allow extending the device photoresponse into the infrared region far below the absorption edge of silicon. Device processing and band structure Silicon microspheres have been obtained by chemical vapour deposition techniques [12] . 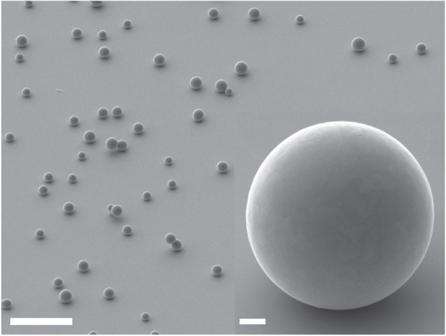Figure 1: Scanning electron microscopy image of polydisperse silicon colloids on a silicon substrate from a bird’s-eye point of view. The inset shows a detailed view of a single sphere, where the polycrystalline nature can be seen on its surface, thanks to grain contrast effects. The scale bars are 20 μm in the general view and 500 nm in the inset. Figure 1 shows a scanning electron microscopy image of several polycrystalline silicon microspheres. The inset of the figure shows a high-magnification image of a single particle, with spherical shape (diameter, d =3.57 μm), where the small silicon nanocrystallites can be appreciated, thanks to grain contrast effects. To develop rectifying junctions in the particles, silicon colloids were synthesized directly onto n -type silicon substrates with an n + -layer implanted on top. The samples were annealed at temperatures between 850 and 1,100 °C, allowing a recrystallisation of the silicon microspheres, an improvement of the substrate–particle electrical contact, and a diffusion of n -type impurities from the substrate into the bottom side of the particles. After that, a very thin (10 nm) indium tin oxide (ITO) conductive transparent layer was sputtered onto the system. The process leaves an ITO-free gap region between the particles and the substrate (see the schematic in Fig. 2 ). At this stage, thousands of ITO/sphere/ n -Si spherical devices, back-connected through the substrate, are obtained. Finally, to test a single device, an all-metallic platinum atomic force microscope (AFM) tip is used to contact on a single sphere. This procedure is appropriate to study the photoresponse of a single sphere, offering a painless and fast way for selecting and contacting the desired device. Figure 1: Scanning electron microscopy image of polydisperse silicon colloids on a silicon substrate from a bird’s-eye point of view. The inset shows a detailed view of a single sphere, where the polycrystalline nature can be seen on its surface, thanks to grain contrast effects. The scale bars are 20 μm in the general view and 500 nm in the inset. 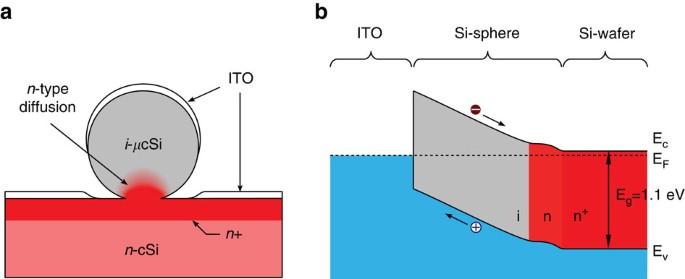Figure 2: Schematic representation of the device structure and band diagram. (a) Basic structure of the device. (b) Band diagram proposal of the device. The direction of carrier separation has been indicated for convenience. Full size image Figure 2: Schematic representation of the device structure and band diagram. ( a ) Basic structure of the device. ( b ) Band diagram proposal of the device. The direction of carrier separation has been indicated for convenience. Full size image During the annealing process, n -type impurities diffuse from the n + substrate into the core of the particle. Considering Fick’s law (and for crystalline silicon), one wouldn’t expect a diffusion length longer than 300 nm for the annealing temperatures and time used. However, since spheres recrystallize at the same time, we cannot discard the possibility that impurities could diffuse much deeper inside the sphere. Therefore, we have two device scenarios. In the first one, the impurities diffuse completely into the whole volume of the silicon sphere. In the second one, the impurities are localised within the sphere near the n + silicon substrate interface. It is agreed that sputtered ITO tends to produce a rectifying structure when deposited over n -type silicon [19] but an ohmic contact when deposited over p -type silicon [20] . Therefore, we can assume that the ITO layer behaves as p -type electrode. Consequently, in the first scenario case, where n -type impurities fill the whole silicon particle and reach the top surface of the microresonator, the rectifying effect would come from the ITO- n Si Schottky junction. However, in the second scenario, where only the bottom part of the sphere is doped, the structure would resemble a PIN diode. In both cases, the charge separation would be very similar. In Fig. 2 , we show the tentative band diagram in this second scenario, that we reckon is the most probable. Electrical characterization and spectral response Single spherical devices, contacted through a conductive AFM tip, where characterized electrically using a precision source measure unit. To record the spectral response of the devices, a tunable monochromatic source was focused on a sphere while measuring the photogenerated short circuit current. The set up is shown schematically in Fig. 3c and a detailed description is given in the Methods section. 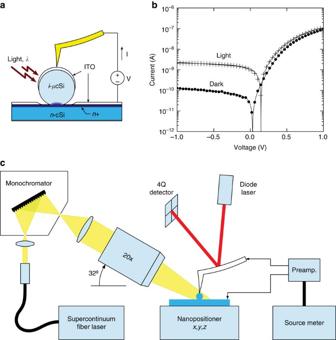Figure 3: Schematic of the measurement set up. (a) Spherical device schematic. Back contact is done through the substrate while front contact is achieved by using a platinum AFM tip. (b) Measured current–voltage, I–V, characteristic of a typical sphere (d=2.9 μm) in dark (dots) and under illumination (crosses) using monochromatic laser light of 990 nm in wavelength. The solid lines correspond to a standard two-diode model fit. (c) Schematic of the set up developed for measuring the spectral response of the spherical devices. The current is measured using a home-made conductive AFM system (see theSupplementary Informationfor more details). A monochromatic tunable source, composed by a supercontinuum laser and a monochromator, is focused on a single sphere at 32° with respect to the sample plane. Figure 3b shows the I–V characteristic of a typical spherical diode ( d =2.9±0.1 μm) under both dark and illumination conditions (see also the Supplementary Fig. 1 ). In darkness, there are three orders of magnitude difference between forward and reverse bias current, a reasonable rectifying behaviour. A small open circuit voltage can be observed, which we attribute to the scattered light from the red laser used for the tip control. Under illumination, both photocurrent and power are generated, demonstrating the capability of the device to work as both detector and micro-power source. The sphere was illuminated with IR monochromatic light at a wavelength of 990 nm, in the absorption edge of silicon, with around 1 sun (1 kW m −2 ) of equivalent intensity, this resonating with a whispering gallery mode of the microcavity. In spite of the small optical absorption of silicon in the infrared, the photodiode exhibits 1±0.1 nA short-circuit current, 0.15±0.02 V open-circuit voltage, and a maximum output power of 42±8 pW with a fill factor of 30%. It corresponds to a non-negligible efficiency value of around (0.6±0.15) %, and an external quantum efficiency (EQE) of (18±5) %. Figure 3: Schematic of the measurement set up. ( a ) Spherical device schematic. Back contact is done through the substrate while front contact is achieved by using a platinum AFM tip. ( b ) Measured current–voltage, I–V, characteristic of a typical sphere ( d =2.9 μm) in dark (dots) and under illumination (crosses) using monochromatic laser light of 990 nm in wavelength. The solid lines correspond to a standard two-diode model fit. ( c ) Schematic of the set up developed for measuring the spectral response of the spherical devices. The current is measured using a home-made conductive AFM system (see the Supplementary Information for more details). A monochromatic tunable source, composed by a supercontinuum laser and a monochromator, is focused on a single sphere at 32° with respect to the sample plane. Full size image The left panel of Fig. 4 , shows the spectral response of the photocurrent in the NIR region for different microcavities whose diameters are 3.9, 3.3, 3.2 and 2.9 μm from top to bottom, respectively. To minimize the influence of both the substrate and the AFM tip on the resonant modes, the impinging laser light was focused on the spheres at an incidence angle of 32° with respect to the substrate plane (see inset in Fig. 4 ). There are several astonishing features in the photocurrent response that are completely different from those of either a planar photodiode or nanowire solar cells so far developed. First, the obtained photoresponse shows very rich spectra with plenty of high- Q resonant peaks. Over the photocurrent background line, which is at least 10 times larger than the dark current level, clusters of narrow resonance peaks appear in a similar manner as the scattering spectra of high order whispering gallery modes in spherical microcavities [21] . Roughly speaking, the photocurrent response at the resonances is boosted about five times over the base line. We will later discuss this point at the light of theory. Also, when the peak position is scaled to the size parameter value α , defined as α =π d / λ , the features appear scaled at about equivalent size parameter values, this being independent of the sphere diameter, d , as expected from the Mie theory (see right panel of Fig. 4 ). However, the photocurrent features show small shifts for different sphere diameter values that we ascribe mainly to the refractive index dispersion appearing in the large spectral zone scanned and the uncertainties in the particles’ size. This is an experimental test of the Mie-like origin of the photocurrent resonances. There are also small differences between the peaks structure coming from different diodes that we ascribe to either the tiny deformation of the spherical shape or to the defects appearing inside the spheres (see the Supplementary Fig. 2 ). Second, as a consequence of the enhanced resonant absorption, the photocurrent response extends far below the band gap of silicon (around 1,150 nm). In fact, these peaks extend beyond the measurement range of the equipment (1,700 nm). Silicon particles are not crystalline but polycrystalline indeed; therefore, the residual defect-connected absorption [22] should be strongly enhanced by the long photon-dwell time at the Mie resonances, extending the photocurrent response well beyond the absorption edge of bulk silicon. The extended photoresponse in the IR region may open the possibility for developing silicon-based photodiodes in the third telecom window (around 1,500 nm of wavelength). 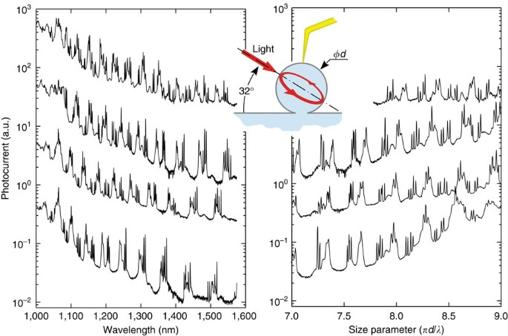Figure 4: Photocurrent spectral response of several devices. Left, spectral response (short-circuit photocurrent) of microcavities with different diameter values of, from top to down, 3.9, 3.3, 3.2 and 2.9 μm. Right, the same spectra of the left side but plotted as a function of the size parameter. The measured curves are vertically shifted for the sake of clarity in both cases. Figure 4: Photocurrent spectral response of several devices. Left, spectral response (short-circuit photocurrent) of microcavities with different diameter values of, from top to down, 3.9, 3.3, 3.2 and 2.9 μm. Right, the same spectra of the left side but plotted as a function of the size parameter. The measured curves are vertically shifted for the sake of clarity in both cases. Full size image Owing to the strong light localization at the high- Q Mie resonances, two-photon absorption process might also come into play. To verify this, we have measured the dependence of the short-circuit photocurrent with the light intensity. We introduced a beam splitter in between the monochromator and the focusing objective and simultaneously monitored the photocurrent and the incident intensity with a power metre. 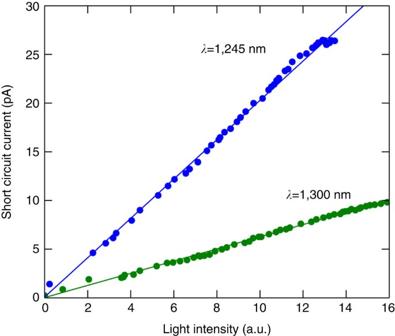Figure 5: Short-circuit current versus the light intensity for two different wavelength values. The blue curve (λ=1,245) was measured in a resonance peak, while the green curve (λ=1,300) was measured off resonance. Figure 5 shows the dependence of the photocurrent with the light intensity at two different wavelength values located on resonance (blue line) and off resonance (green line). In both cases, the dependence is linear, suggesting that the photocurrent enhancement is actually due to the increased dwelling time of photons at the resonances. Figure 5: Short-circuit current versus the light intensity for two different wavelength values. The blue curve ( λ =1,245) was measured in a resonance peak, while the green curve ( λ =1,300) was measured off resonance. Full size image In the previous sections, we have provided experimental evidence of the resonance enhancement of IR absorption in the spherical cavities. A realistic calculation of either the absorption efficiency or the photocurrent response of the devices is beyond the goal of this paper and it would require a precise knowledge of the different parameters involved. The devices’ response is very sensitive to many unknown parameters, making it very difficult to obtain an accurate fit to the measured spectra. For instance, the absorption tail below the gap strongly depends on the polycrystalline character of the optical cavity, an unknown parameter in the present state of the art, which would determine the Q values of the photocurrent peaks. More importantly, the Mie resonances and their clustered structure strongly depend on the precise device topology. The effect of the substrate and tip, the void-defects and inhomogeneities randomly appearing in the interior of the spheres (see Supplementary Fig. 2 ), and even the slightest warping of the spheres, all them have a profound impact on the spectral response. In Supplementary Note 1 and Supplementary Figs 3–6 , we show the strong influence of these parameters at the light of different theoretical models. Although fitting the experimental data is difficult, we can easily estimate the potentiality of the device by analysing the relationship between the Q value of the photocurrent peaks and the maximum absorption efficiency expected for the device in the infrared region. The absorption efficiency in a typically high- Q resonance, that is, at the peak wavelength of a Mie resonance, is proportional to the Q value of the mode. The higher the Q value, the longer the dwell time of photons within the cavity, this leading to a larger absorption probability. An upper bound for the resonant absorption enhancement, A , of a free standing sphere can be defined as the ratio between the time spent by a photon in the cavity over the time needed to travel a distance equivalent to the diameter of the sphere, , where n is the refractive index of silicon, d , is the diameter of the sphere, and λ is the wavelength of light. However, an extra ½ factor must be added to account for the effect of the substrate (half of the modes are damped by the substrate). The enhancement A /2 takes a value around Q /100 over the wavelength range of measurements and for an average particle size of 3 μm. As the top Q values measured lay around 10 3 , a maximum photocurrent enhancement of about ten over the bottom line is expected, which is of the same order of magnitude of experimental results. Overall, at the high- Q resonant peaks, well below the absorption edge of silicon, we have observed EQE values exceeding (1±0.25) % at wavelengths of up to 1,500 nm, a remarkable value for such a tiny particle in a spectral region where bulk silicon shows a negligible absorption. Devices with larger Q factor resonances, or simply devices with tuned particle size, would harvest light more efficiently in the infrared region. Furthermore, the combined absorption of multiple nearby particles, featuring multiple scattering effects, could lead to even higher efficiencies and broader, smoother spectral responses. In conclusion, we have developed a rectifying device in a polysilicon spherical Mie resonator. The photocurrent spectra show strong resonances mimicking the resonant absorption process of a Mie resonator at wavelength values much below the typical absorption edge of silicon. This may open the door for developing all silicon spherical photodiodes and photovoltaic cells with a useful spectral response in the near infrared region. Sample fabrication The following is a detailed description of the technological steps used to fabricate the devices. The starting material was 4-inch, single-side-polished, ‹100› oriented, n -type crystalline Si wafers with a resistivity of 1 Ωcm. On both sides of the wafers, we diffused an n + layer following a standard process and, then, cut them into sample stripes of 1.5 × 5 cm 2 . A single sample stripe was used for each single synthesis process. Before every CVD synthesis reaction, the remaining silicon from the previous process is removed from the reactor’s inner walls with a hot TMAH (25%) solution followed by a standard RCA two-steps cleaning process. The reactor is thoroughly rinsed with deionized water after every cleaning step and let to dry. We remove the native oxide from the sample with a short dip (10 s.) in HF (5%) just before introducing it into the reactor. When the reactor vacuum reaches a level below 10 −6 mbar, we fill it with a low pressure, namely about 20 kPa, of disilane (Si 2 H 6 ) gas and close it. The reactor is then introduced in an oven at a temperature between 400 and 600 °C for 30 min., decomposing the disilane gas and producing the silicon particles, which fall over the sample as a kind of soot. Finally, the exhaust gases are pumped out the reactor before retrieving the sample. These conditions of temperature and pressure produce a monolayer of isolated amorphous spheres, with an average size of 3 μm. Also, a thin epitaxial layer of silicon grows in a conformal manner on the substrate and around the spheres, thus covering the bottom of the sphere in close contact to the silicon substrate. It results in the formation of a neck between the substrate and the silicon particle, facilitating the electrical connection between them (see Fig. 1 and the Supplementary Fig. 2 ). Once the silicon particles were synthesized, we annealed them in a horizontal tube furnace for 1 h at temperatures between 850 and 1,100 °C in pure N 2 atmosphere at ambient pressure. In this way, amorphous silicon spheres are converted into polycrystalline ones, improving the sphere–substrate contact, and allowing n -type impurities to diffuse into the sphere. Before the annealing process, the samples were cleaved in halves (0.7 × 5 cm stripes), so that the number of samples was doubled, rinsed in deionized water and dipped in HF (5%) to remove the native oxide. After all the different annealing processes were performed, all samples were dipped in HF once more to remove any trace of silicon dioxide and introduced all of them in the sputtering chamber. Ten nanometres of ITO was sputtered over all of them at once, ensuring the same ITO layer for all silicon microcavities. A bare polished silicon witness was used to control the ITO layer thickness. Finally, a small portion of the samples (1 cm) is cleaved and glued to a standard AFM metallic disc using silver conductive adhesive so that the samples can be handled and contacted through the disk. Notice that the process preserves the surface of the samples, thus avoiding any contact with both the substrate and the particles. We have fabricated nearly 100 samples, most of them devoted to tune the sphere synthesis process and to increase the sphere’s quality. For the present work, we have processed 16 different samples covering different parameters, namely the doping level of the substrate (with/without n + diffused layer) and the annealing temperature (from 850 to 1,200 °C in steps of 50 °C). Experimental set up Figure 3c shows a schematic representation of the system developed for measuring the spectral response of a single spherical device. It is composed basically by two subsystems: a tunable monochromatic source used for excitation; and a home-made conductive Atomic Force Microscope (c-AFM) used to measure both, the I–V characteristic and the photocurrent response of a single particle. The tunable monochromatic source is accomplished by a Fianium SC400 supercontinuum fibre laser source (400–2,400 nm) coupled to a Horiba Triax 190 monochromator equipped with a 900 l mm −1 grating. With this combination, we achieve a spectral resolution of 0.5 nm in the wavelength range 900–1,700 nm. The laser beam is focused on a sphere, through a × 20 objective, at an incidence angle of 32° with respect to the substrate plane. The objective is slightly out of focus so that it easily allows us to illuminate the region where the device is located. The home-made c-AFM was designed with the goal of being accessible for the optical elements around, specially the optical objectives. We used M Plan Apo NIR objectives from Mitutoyo, as they provided optimum performance in the wavelength range of interest and the long working distance needed for the set up. The samples are attached to a long-range x , y , z nanopositioner while the conductive probe is held fixed, it’s depletion being constantly monitored by the signal of a reflected laser detected by a four-quadrant detector. Solid metallic (Pt) conductive probes from Rocky Mountain, with a spring constant of 18 N m −1 , provided optimum contact and the right endurance through the spectral response experiments. An additional optical objective (not shown in the schematic) permits top-view inspection of the tip and the sample. Finally, current/voltage measurements are acquired using a Keithley 6430 source meter with a remote preamplifier that allows both voltage and current sourcing/measuring with high sensitivity. During a standard I(V) curve acquisition, voltage is sourced while current is measured. During spectral measurements, the photogenerated short-circuit current (V=0) is measured while we scan the spectral region of interest with the monochromatic source. Reproducibility and measurement error treatment In total, we prepared 16 samples specifically for this work but many more were prepared to optimize the particle synthesis and also for developing the device. Repeatability of results are excellent in the sense that no matter what sample or particle we measure, we obtain a spectrum with resonance peaks extending in the IR as long as the sphere has not been ripped off the surface. The particular spectrum depends, obviously, on the size and quality of the selected sphere, but subsequent measurements of the same particle yield the same spectrum. Even different particles from the same sample give spectra that scales well with the size parameter, as shown in the Fig. 4 . Furthermore, new samples fabricated afterwards following the same process provided similar spectra. Electrical voltages/currents are sourced/measured with excellent accuracy and are well above the resolution of the instrument. For instance, the instrument is capable of measuring currents below a femto-ampere, but we normally measure current in the range 10 pA–1 nA. Measured current, however, is sensitive to the tip–sphere contact. Slight changes in the spectra can be appreciated when changing the AFM tip or when changing the tip pressure. Notice that this does not change the spectra shape but scales them. We use stiff solid-platinum AFM tips applying a high pressure, which provides a robust contact but, nevertheless, it is safe to consider a 10% uncertainty in the photocurrent absolute values due to the tip contact changes. The larger uncertainties in the estimation of the EQE or the efficiency, concerns the difficulty in determining the illumination intensity impinging on the particles. Although the total light intensity exiting the objective can be precisely measured with a power meter, we are not able to precisely determine the area shined. To estimate it, we try to view the illuminated area with the aid of a rough surface, and used this value to estimate de EQE and the efficiency values reported on the main text. With this method, we estimated the diameter of the illuminated spot to be within 150–200 μm, resulting in a device efficiency error of ±30% at the wavelength values of the Mie resonances. How to cite this article: Garín, M. et al. All-Silicon spherical-Mie-resonator photodiode with spectral response in the infrared region. Nat. Commun. 5:3440 doi: 10.1038/ncomms4440 (2014).